Toxicity modelling of Plk1-targeted therapies in genetically engineered mice and cultured primary mammalian cells High attrition rates of novel anti-cancer drugs highlight the need for improved models to predict toxicity. Although polo-like kinase 1 (Plk1) inhibitors are attractive candidates for drug development, the role of Plk1 in primary cells remains widely unexplored. Therefore, we evaluated the utility of an RNA interference-based model to assess responses to an inducible knockdown (iKD) of Plk1 in adult mice. Here we show that Plk1 silencing can be achieved in several organs, although adverse events are rare. We compared responses in Plk1-iKD mice with those in primary cells kept under controlled culture conditions. In contrast to the addiction of many cancer cell lines to the non-oncogene Plk1 , the primary cells' proliferation, spindle assembly and apoptosis exhibit only a low dependency on Plk1. Responses to Plk1-depletion, both in cultured primary cells and in our iKD-mouse model, correspond well and thus provide the basis for using validated iKD mice in predicting responses to therapeutic interventions. Although mice and humans are different, genetically engineered mouse models (GEMMs) in cancer research faithfully reflect many of the fundamental traits of human cancer, which suggests that they are valuable tools for understanding the biology of tumour development and growth [1] . In conventional knockouts, the loss of a vital gene often leads to embryonic lethality or severe developmental abnormalities, which obscure the study of potential functions in the adult organism. To circumvent these obstacles, conditional genetic engineering technologies have been developed to control gene expression spatially and temporally. One current strategy is controlled expression of site-specific recombinases to delete the specific gene of interest [2] . Alternatively, loss-of-function studies use sequence-specific RNA interference (RNAi)-based approaches to silence the expression of target genes [3] ; this method often recapitulates the clinical effects of anti-cancer drugs better than transgenic models with null phenotypes because under clinical conditions, specific cancer targets are only partially inhibited and are often time-limited depending on the applied drug scheduling [2] , [4] . Anti-mitotic drugs that inhibit microtubule dynamics have been successful in the treatment of cancer [5] , [6] . Still, their effectiveness is limited by two critical aspects: resistance and toxicity (myelosuppression and neuropathies). In efforts to avoid adverse side effects, small molecule inhibitors were developed to target the critical regulators of mitosis, such as polo-like kinase 1 (Plk1), that are overexpressed in a wide range of tumour types [7] , [8] , [9] , [10] , [11] . In vertebrate cells, Plk1 has been implicated in multiple steps of mitotic progression including the activation of Cdk1/cyclin B1 (ref. 12 ), centrosome maturation, release of cohesion from chromosomes, activation of the anaphase-promoting complex/cyclosome, formation of bipolar spindles and the regulation of the spindle assembly checkpoint (SAC) [8] , [13] , [14] , [15] . Inhibitors targeting Plk1 have recently entered the clinic [16] . Because the role of Plk1 in primary normal cells remains widely unexplored and homozygous Plk1 null-mice are embryonic lethal [17] , in this study we generated an inducible RNAi-based GEMM as a tool to determine the function of mammalian Plk1 in adult mice and to monitor putative adverse events. We explored the effects of Plk1 gene dosage on the mitotic activity and induction of apoptosis in primary cells in vivo and in vitro . Our results suggest that transgenic inducible RNAi technology is helpful for modelling the function of pharmacologically relevant targets in adult mice. Examining Plk1 knockdown in embryonic stem cells The first aim of this study was to model the function of Plk1 in adult mice using an inducible RNAi technique. We tested 18 small hairpin RNA (shRNA) constructs targeting murine Plk1 at different sites in NIH3T3 and RENCA cells. Plk1 silencing was induced by various shRNAs, which suggests that the effect was not due to the off-target effects from a single-RNAi site. We selected the shRNA-Plk1/1473 because it knocked down Plk1 mRNA by more than 70% ( Supplementary Table S1 ). To prevent the chromosomal positional effects associated with the random nature of transgene integration, we inserted a cassette for shRNA expression into the well-characterized euchromatic locus Rosa26. The shRNA sequence Plk1/1473 was placed under the control of our previously generated inducible H1 promoter along with a genetic element for the constitutive expression of the codon-optimized tetracycline repressor protein (itetR) [18] , [19] , [20] , [21] ( Supplementary Fig. S1a ). The standard transfection procedures using this exchange vector were followed by the recombinase-mediated integration, which resulted in more than 90% positive embryonic stem (ES) cell clones ( Supplementary Fig. S1b–d ). The doxycycline (Dox)-dependent expression of shPlk1, followed by the processing of siPlk1 in transgenic ES clones, was confirmed by stem–loop reverse transcription–PCR (RT–PCR; Supplementary Fig. S1e ). The 75–80% Dox-induced reduction of Plk1 mRNA and the 80–90% protein reduction were determined ( Supplementary Fig. S1f,g ). The constitutive expression of itetR was confirmed ( Supplementary Fig. S1g ). Thus, on Dox-treatment of the ES cells, the shRNA cassette was integrated into the Rosa26 locus to allow inducible regulation of Plk1 expression or Plk1-inducible knockdown (iKD). In Plk1-depleted ES cells the levels of other Plk members (Plk2-4) remained nearly unchanged supporting the specificity of our Plk1-targeted RNAi-approach ( Supplementary Fig. S1h ). The generation and knockdown analysis of Plk1-iKD mice Mice harbouring a heterozygous insertion of the shRNA (Plk1-iKD) were developed by tetraploid embryo complementation from the recombinant ES cells [20] . Analysis of the adult tissues before Dox-treatment confirmed Plk1 expression in tissues that contained an elevated percentage of proliferating cells, including those of the testis, thymus and spleen ( Fig. 1a,b ). Next, we verified the presence of the shRNA cassette in the tail clips of Plk1-iKD mice by PCR ( Fig. 1c ) and determined the efficiency of the shRNA cassette by monitoring the activity of the cytomegalovirus-enhancer/β-actin (CAG)-itetR system. The CAG-driven expression of itetR was detected in all tested tissues ( Fig. 1d ). The subsequent knockdown analyses focused on adult tissues of wild-type (wt) mice that expressed Plk1 at above background levels. Following 6 weeks of Dox-treatment, the quantitative reverse transcription (qRT–PCR) analysis revealed a substantial depletion of the Plk1 mRNA in various organs of Dox-treated Plk1-iKD mice (testis: 86% reduction; bone marrow: 72%; and spleen: 60%) compared with the mRNA levels in Dox-treated wt mice ( Fig. 1e ). Analysis of the Plk1 protein expression confirmed efficient silencing in various murine organs (spleen, testis, ovary, stomach and colon) with residual levels (<10–20%; Fig. 1d ). The expression of Plk3, which was previously shown to have overlapping functions with Plk1 in a yeast complementation assay [22] , [23] , in the tissues of Dox-treated Plk1-iKD mice did not differ markedly compared with those in wt mice ( Fig. 1d ). 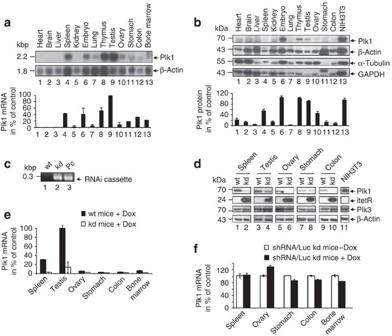Figure 1: Analysis of RNAi-based depletion of Plk1 in the tissues of adult transgenic mice. (a) Poly(A)+mRNA, isolated from the tissues of untreated adult mice and from 14-day-old embryos, was analysed by northern blot using32P-labelled probes for Plk1 and β-actin, the loading control. Autoradiography was performed at 16 h. The bar graph represents the Plk1 mRNA expression standardized to the β-actin expression (means±s.d.,n=5, for each tissue). (b) Total cellular protein prepared from the indicated tissues of untreated adult mice, embryos and NIH3T3 cells were separated by SDS–PAGE and immunoblotted for anti-Plk1, anti-β-actin, α-tubulin and GAPDH as loading controls (means±s.d.,n=5, for each tissue). (c) PCR of mouse genomic DNA (tail clip) from wild-type (wt) mice, Plk1-iKD mice (kd) and template DNA as the positive control (pc) are presented. (d) Total cellular protein was prepared from the indicated tissues of Dox-treated adult Plk1-iKD and wt mice and separated by SDS–PAGE for anti-Plk1, -itetR, -Plk3 and -β-actin immunoblotting analyses. (e) Plk1 mRNA levels in the tissues of Dox-treated Plk1-iKD and wt mice relative to the Plk1 mRNA levels in the testis of untreated animals (100%), which was the tissue with the highest Plk1 mRNA expression, are shown (means±s.d.,n=5, for each tissue). (f) Relative Plk1 mRNA levels in the tissues of Dox-treated Luc-iKD (Luc-iKD +Dox) animals are compared with the levels in untreated Luc-iKD animals (Luc-iKD -Dox; means±s.d.,n=3, for each tissue). Figure 1: Analysis of RNAi-based depletion of Plk1 in the tissues of adult transgenic mice. ( a ) Poly(A) + mRNA, isolated from the tissues of untreated adult mice and from 14-day-old embryos, was analysed by northern blot using 32 P-labelled probes for Plk1 and β-actin, the loading control. Autoradiography was performed at 16 h. The bar graph represents the Plk1 mRNA expression standardized to the β-actin expression (means±s.d., n =5, for each tissue). ( b ) Total cellular protein prepared from the indicated tissues of untreated adult mice, embryos and NIH3T3 cells were separated by SDS–PAGE and immunoblotted for anti-Plk1, anti-β-actin, α-tubulin and GAPDH as loading controls (means±s.d., n =5, for each tissue). ( c ) PCR of mouse genomic DNA (tail clip) from wild-type (wt) mice, Plk1-iKD mice (kd) and template DNA as the positive control (pc) are presented. ( d ) Total cellular protein was prepared from the indicated tissues of Dox-treated adult Plk1-iKD and wt mice and separated by SDS–PAGE for anti-Plk1, -itetR, -Plk3 and -β-actin immunoblotting analyses. ( e ) Plk1 mRNA levels in the tissues of Dox-treated Plk1-iKD and wt mice relative to the Plk1 mRNA levels in the testis of untreated animals (100%), which was the tissue with the highest Plk1 mRNA expression, are shown (means±s.d., n =5, for each tissue). ( f ) Relative Plk1 mRNA levels in the tissues of Dox-treated Luc-iKD (Luc-iKD +Dox) animals are compared with the levels in untreated Luc-iKD animals (Luc-iKD -Dox; means±s.d., n =3, for each tissue). Full size image The generation and knockdown analysis of luciferase-iKD mice A sequence against the firefly luciferase ( Luc ) gene served as a control siRNA that had no significant homology to any known murine genes, to establish a second iKD-mouse model to control the toxicity of siRNA expression under the Dox-inducible promoter. Luc-iKD mice were generated harbouring a CAG-itetR/H1tetO-shRNA/Luc-cassette inserted into the rosa26 locus according to the procedure described above. We could not detect any significant changes between the Luc-iKD and control mice (both Dox-treated) in terms of the transcript levels of Plk1 ( Fig. 1f ) or other control genes ( Cdk1, MAPK1, histone H1 ) in various tissues. This observation supports the notion that the Dox-inducible Pol III RNAi system used for our GEMM only marginally affects the expression of certain non-target genes. Phenotypic analysis of Plk1-iKD mice Plk1-iKD mice treated with Dox for 6 weeks underwent a thorough phenotypic analysis at the German Mouse Clinic (GMC), which included several hundred parameters in dysmorphology, neurology, clinical chemistry, immunology, allergy, steroid metabolism, cardiovascular function, nociception, energy metabolism and pathology [24] . Selected parameters of the phenotypic analysis relevant to the function of Plk1 include the following: the complete morphological analysis did not reveal histological differences between the organs of Dox-treated Plk1-iKD mice and those of control animals ( Supplementary Fig. S2a ). Our GMC metabolic screening programme provided a comparative analysis of bioenergetic parameters in the transgenic mice. The mechanisms that lead to disturbances in body weight regulation and energy metabolism were examined, including food consumption, energy uptake, faeces production, energy content in the faeces and metabolized energy, which all remained unchanged. Despite their low values of assimilated energy, Dox-treated male Plk1-iKD mice had a significantly increased body mass and rectal temperature compared with those of control animals ( Supplementary Table S2 ). Given that the function of Plk1 is critical for mitosis, we examined the proliferative activity in iKD-mice: the proliferation index was moderately reduced in only the mucosal folds of the large intestines and in the ovarian follicles ( Fig. 2a,b , Supplementary Tables S3 and S4 ). A significant induction of apoptosis as determined by the TdT-mediated dUTP nick end labelling assay was not apparent in murine tissues. Considering that the Drosophila counterpart of Plk1 , polo , is crucial for normal spermatogenesis in Drosophila [25] , we examined the testes of Plk1-iKD mice that exhibited a strong reduction (86%) in Plk1 levels. The weight of the testis from the Dox-treated Plk1-iKD mice was not significantly different from that of the control animals (0.095 versus 0.0985 g, P =0.206), indicating normal spermatogenesis. Within the seminiferous epithelium, spermatogenesis proceeds from the basal to adluminal layers; thus, the mitotically active spermatogonia are located at the periphery of the epithelium ( Fig. 2c ). A morphometric analysis was performed on tubules that were in stages VII/VIII of the seminiferous epithelial cycle; these tubules exhibited the highest number of Ki-67-positive spermatogonia corresponding to the stage-specific pattern of murine spermatogonial mitotic activity [26] , [27] . The percentage of Ki-67-positive spermatogonia in control (87.3%) and Plk1-iKD mice (87.7%) was similar further suggesting that normal spermatogenesis occurred in both groups ( Fig. 2c ). Myelosuppression is a common side effect associated with the therapeutic use of anti-mitotic drugs such as taxanes [5] . To elucidate whether the silencing of Plk1 causes similar adverse events, the GMC haematology and immunology screen focused on putative haematological changes. Neither the total white blood cell count nor the number of erythrocytes (red blood cells) or platelets was significantly reduced in iKD mice. Although the proportions of B cells and NK cells (% of CD45+ cells) were slightly increased, the granulocyte compartment was reduced in the Dox-treated iKD mice compared with those in the controls ( Supplementary Table S5 ). The negative linear correlation between the frequencies of granulocytes and B cells is a common observation in wt mice and reflects physiological regulation mechanisms [28] . As the proportion of granulocytes in the Dox-treated wt mice increased compared with that in the untreated controls and iKD mice, the Dox-treatment itself might have influenced the proportions of leukocyte subsets in the peripheral blood. Because granulocyte proportions were still within the physiological range and the total white blood cell count was not reduced, we found no indication of neutropenia. Thus, after 6 weeks of Dox-treatment, we observed no signs of bone marrow suppression in Plk1-iKD mice. Among the 21 parameters identified in the clinical–chemical plasma screen, substantial differences were detected only in serum ferritin, which has been implicated in the regulation of hematopoiesis [29] . Ferritin values were reduced in Plk1-iKD mice (male control: 37.4±3.1 ng ml −1 ; female control: 37.9±2.0 ng ml −1 ; male transgenic: 10.2±1.4 ng ml −1 , female transgenic: 13.8±1.0 ng ml −1 , P <0.001), suggesting an iron deficiency [29] ( Fig. 2d ). However, the mice showed no signs of iron deficiency, anaemia, except that they had a slightly increased anisocytosis (red blood cell distribution width RDW) in the peripheral blood cell count. Overall, the examination indicated that during efficient Plk1 depletion (>80%) in the different organs, the low levels of any remaining Plk1 were sufficient to maintain cellular proliferation, spermatogenesis and hematopoiesis in adult mice. 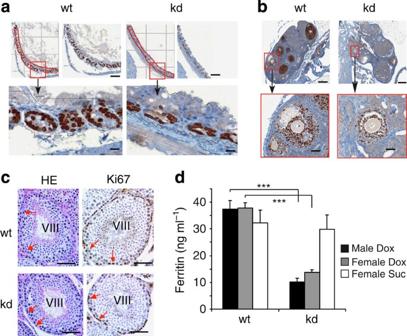Figure 2: Phenotypic comparison of Plk1-iKD and wt mice. (a–c) Representative examples are shown. (a) Determination of the proliferation index in the mucosal folds of the large intestine: Ki-67-stained cells in the crypts of the transverse mucosal folds of the large intestine of a wt and a Plk1-iKD mouse. Sections are shown at two magnifications. Upper scale bars, 500 μm, lower scale bars, 50 μm. (b) Determination of the proliferation index of the ovarian follicles: Ki-67-stained cells of an ovarian follicle of a wt and of a Plk1-iKD mouse. To calculate the proliferative index in the cyclic ovary, follicles of similar sizes were selected (red boxes). Sections are shown at two magnifications. Upper scale bars, 500 μm, lower scale bars 50 μm. (c) Seminiferous tubules (stage VIII) in the testis of wt and iKD animals (primary magnification: ×20, arrows point to spermatogonia) were Bouin fixed, stained with hematoxylin/eosin or formalin fixed and stained for Ki-67 immunohistochemistry (brown nuclei of spermatogonia) with hematoxylin counterstaining. Scale bar, 50 μm. (d) Ferritin values were determined using an AU400 autoanalyzer (Olympus) in female and male Plk1-iKD mice and a sucrose-treated control group, which were all treated with Dox (means±s.e.m.,n=3, for each sample). ***P<0.001, Student'st-test, unpaired and two-tailed. Figure 2: Phenotypic comparison of Plk1-iKD and wt mice. ( a – c ) Representative examples are shown. ( a ) Determination of the proliferation index in the mucosal folds of the large intestine: Ki-67-stained cells in the crypts of the transverse mucosal folds of the large intestine of a wt and a Plk1-iKD mouse. Sections are shown at two magnifications. Upper scale bars, 500 μm, lower scale bars, 50 μm. ( b ) Determination of the proliferation index of the ovarian follicles: Ki-67-stained cells of an ovarian follicle of a wt and of a Plk1-iKD mouse. To calculate the proliferative index in the cyclic ovary, follicles of similar sizes were selected (red boxes). Sections are shown at two magnifications. Upper scale bars, 500 μm, lower scale bars 50 μm. ( c ) Seminiferous tubules (stage VIII) in the testis of wt and iKD animals (primary magnification: ×20, arrows point to spermatogonia) were Bouin fixed, stained with hematoxylin/eosin or formalin fixed and stained for Ki-67 immunohistochemistry (brown nuclei of spermatogonia) with hematoxylin counterstaining. Scale bar, 50 μm. ( d ) Ferritin values were determined using an AU400 autoanalyzer (Olympus) in female and male Plk1-iKD mice and a sucrose-treated control group, which were all treated with Dox (means±s.e.m., n =3, for each sample). *** P <0.001, Student's t -test, unpaired and two-tailed. Full size image The long-term Dox-treatment (>30 months) induced only a moderately reduced survival rate comparing iKD and wt mice ( Supplementary Fig. S2b ). To investigate the genomic stability of the Plk1-iKD-cassette, we performed a genotyping of a random collection of littermates. Considering that the first Plk1-iKD ES cells and mice were generated between June 2006 and August 2006, the presence of the iKD-cassette in mice of different ages in March 2011 demonstrated the stability of the iKD for a period of 4.5–5 years (≥10 generations; Supplementary Fig. S2c ). Moreover, the western blot analysis of splenocytes provided evidence for the long-term functionality of the iKD-cassette by showing stable itetR-expression and Dox-inducible depletion of Plk1 ( Supplementary Fig. S2d ). Analysis of Plk1-depleted mammalian cells in culture Next, to determine whether the Plk1-iKD mouse model recapitulates the cellular dependency of primary mammalian cells on Plk1, we examined the effects of gradual Plk1 depletion on the proliferation, cell-cycle progression and apoptosis of mammalian cells under controlled culture conditions. First, we tested the proliferative activity of different iKD mouse embryonic fibroblasts MEF clones ( Fig. 3a ). The Dox concentration (0–80 μg ml −1 ) and the Plk1 protein levels were inversely correlated ( Fig. 3a ). Massive Plk1 depletion (90–95% reduction) with 80 μg ml −1 Dox for 96 h had only a minor impact on the proliferative activity of different iKD MEF clones compared with the wt MEFs (MEF-wt: 12% reduction in proliferative activity, P =0.04; MEF-kd12: 2% reduction, P =0.71; MEF-kd17: 12% reduction, P =0.25; and MEF-kd18: 16% reduction, P =0.24; Fig. 3a ). The gradual depletion of Plk1 in different MEF clones did not alter endogenous levels of Plk3 ( Fig. 3a ). 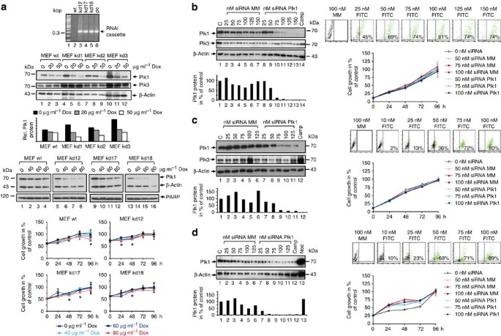Figure 3: Correlation ofPlk1silencing and the proliferative activity of primary mammalian cells. (Upper) (a) PCR of mouse genomic DNA isolated from MEF derived from wild-type (wt) mice, different Plk1-iKD (kd) clones (kd12, 17, 18) and a template DNA as the positive control (pc) are shown. (Middle) Western blot analysis of Plk1 and Plk3 expression in different MEF clones (wt, kd) at increasing Dox concentrations is shown. (Lower) Western blot analysis of Plk1 expression and proliferation of different MEF clones (wt, kd) at increasing Dox concentrations (0–80 μg ml−1) is shown. For standardization, β-actin expression was chosen. The uptake of fluorescein-labelled Plk1 siRNA, Plk1 mRNA depletion and proliferative activity of primary human cells (b) HUVEC, (c) fibroblasts and (d) keratinocytes are shown. (Right) FACS analysis of control cells (that is, incubated with Gene Silencer and non-labelled siRNA MM) and fluorescein-labelled siRNA-transfected cells. The concentration of the Plk1 siRNA is indicated at the top of each panel. Transfections were conducted for 6 h. The intensity of the fluorescence, which represents the uptake of fluorescein-labelled Plk1 siRNA, is indicated in the lower right corner. (Left) The western blot analysis of the Plk1 and the Plk3 protein was conducted 24 h after transfection of the primary human cells with Plk1 siRNA and MM siRNA at the indicated concentrations. β-Actin served as a loading control. Camptothecin (Camp) and/or nocodazole (Noc) controls were included. Plk1 protein expression in primary cells (HUVEC, fibroblasts, keratinocytes) was standardized to the expression of β-actin and is relative to the level of Plk1 in untreated cells (100%). (Right) Proliferative activity of primary cells at different siRNA concentrations (0–100 nM; means±s.d.,n=3, for each time point). *P<0.05, Student'st-test, unpaired and two-tailed. Figure 3: Correlation of Plk1 silencing and the proliferative activity of primary mammalian cells. (Upper) ( a ) PCR of mouse genomic DNA isolated from MEF derived from wild-type (wt) mice, different Plk1-iKD (kd) clones (kd12, 17, 18) and a template DNA as the positive control (pc) are shown. (Middle) Western blot analysis of Plk1 and Plk3 expression in different MEF clones (wt, kd) at increasing Dox concentrations is shown. (Lower) Western blot analysis of Plk1 expression and proliferation of different MEF clones (wt, kd) at increasing Dox concentrations (0–80 μg ml −1 ) is shown. For standardization, β-actin expression was chosen. The uptake of fluorescein-labelled Plk1 siRNA, Plk1 mRNA depletion and proliferative activity of primary human cells ( b ) HUVEC, ( c ) fibroblasts and ( d ) keratinocytes are shown. (Right) FACS analysis of control cells (that is, incubated with Gene Silencer and non-labelled siRNA MM) and fluorescein-labelled siRNA-transfected cells. The concentration of the Plk1 siRNA is indicated at the top of each panel. Transfections were conducted for 6 h. The intensity of the fluorescence, which represents the uptake of fluorescein-labelled Plk1 siRNA, is indicated in the lower right corner. (Left) The western blot analysis of the Plk1 and the Plk3 protein was conducted 24 h after transfection of the primary human cells with Plk1 siRNA and MM siRNA at the indicated concentrations. β-Actin served as a loading control. Camptothecin (Camp) and/or nocodazole (Noc) controls were included. Plk1 protein expression in primary cells (HUVEC, fibroblasts, keratinocytes) was standardized to the expression of β-actin and is relative to the level of Plk1 in untreated cells (100%). (Right) Proliferative activity of primary cells at different siRNA concentrations (0–100 nM; means±s.d., n =3, for each time point). * P <0.05, Student's t -test, unpaired and two-tailed. Full size image As a surrogate for the potential use of Plk1-specific drugs, we depleted Plk1 in human cells of different origins (human umbilical vein endothelial cells (HUVEC), fibroblasts and keratinocytes) by using our previously tested Plk1-specific siRNA [30] , [31] , [32] , [33] . First, we determined the transfection efficiency of the HUVEC using fluorescein-labelled siRNAs by FACS analysis. Using a range of siRNA concentrations (25–150 nM), we measured the uptake of labelled siRNA to be between 45 and 74% ( Fig. 3b ), which was followed by a pronounced reduction of Plk1 protein levels compared with a mismatch (MM) siRNA control ( Fig. 3b ). Despite efficient depletion of the Plk1 protein (>90%), the growth properties of HUVEC did not vary significantly compared with siRNA MM-treated cells (HUVEC: 100 nM siRNA, reduction 6.2% at 96 h, P =0.11, Student's t -test; Fig. 3b ). Silencing of Plk1 did not alter endogenous levels of Plk3 in HUVEC and fibroblasts ( Fig. 3b,c ). In addition, the depletion of Plk1 in human fibroblasts (≥90%) and keratinocytes (>95%) did not significantly inhibit their proliferative activity (fibroblasts: 100 nM siRNA, reduction 0.8% at 96 h, P =0.89; keratinocytes: 100 nM siRNA, no reduction at 96 h, P =0.11, Student's t -test; Fig. 3c,d ). In contrast, human Plk1-depeleted cancer cell lines of different organ origins (cervix, colon, breast, ovary and kidney) showed statistically significant dose-dependent reductions in growth 96 h after transfection compared with that of the siRNA MM-transfected control cells (HeLa: 5 nM siRNA, 82% reduction, P <0.001; SW480: 5 nM siRNA, 66%, P =0.02; MDA-MB-231: 5 nM siRNA, 55%, P =0.02; SK-OV-3: 5 nM siRNA, 46%, P =0.03; 293T: 5 nM siRNA, 51%, P =0.007, Student's t -test; Supplementary Fig. S3a–e ). In summary, although the half-maximal depletion of the Plk1 protein (iKD50 Plk1− ) inhibited the growth of the tested cancer cells by 46–82%, the inhibitory effect in primary cells was <5% ( Table 1 ), which mirrors previous observations in Plk1-iKD mice and supports the model that low Plk1 levels can maintain nearly normal proliferative activity in primary mammalian cells. Table 1 The effect of Plk1 silencing on the proliferation and apoptosis of cancer cells and primary normal cells. Full size table Analysis of the mitotic progression of Plk1-depleted cells Although siRNA MM-transfected cells (HeLa, SW480) regained 2 n content after 15–18 h, the majority of Plk1-depleted cells did not complete their cell divisions ( Supplementary Fig. S4a ). The accumulation of phospho-histone H3 (pHH3(S10)) and the anaphase-promoting complex/cyclosome target cyclin B1 indicate a Plk1 depletion-induced G 2 /M-arrest ( Supplementary Fig. S4b ). Dephosphorylation of p-Cdk1(T14/Y15) by Plk1-activated Cdc25C [34] was delayed by several hours in the Plk1-depleted SW480 cells ( Supplementary Fig. S4b ). The accumulation of Emi1, Securin and pHH3(S10) provided further evidence for the mitotic arrest of Plk1-depleted SW480 cells ( Supplementary Fig. S4b ). The FACS analysis also revealed a pronounced increase in the number of cells in the G 2 /M phase (HeLa: 11→68%, 518% increase; and SW480: 24→48%, 100% increase; Supplementary Fig. S4a ). In contrast, at 24 and 48 h post transfection, the analysis of primary cells showed only a moderate increase in G 2 /M compared with siRNA MM-transfected cells (24 h: HUVEC 100 nM: 27→33%, 22% increase; fibroblasts 100 nM 16→32%, 100% increase; and keratinocytes: 16→20%; 25% increase; Fig. 4a–c ). 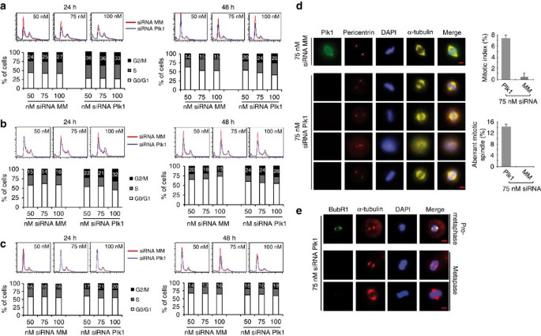Figure 4: Effect ofPlk1silencing on the cell-cycle distribution of primary mammalian cells. Primary cells (a) HUVEC and (b) fibroblasts and (c) keratinocytes were transfected with siRNA MM or siRNA Plk1 at different concentrations (50–100 nM) and analysed by FACS at 24 and 48 h. Representative histograms and the quantification of the cell-cycle analysis are shown. (d) Keratinocytes were labelled using Plk1, pericentrin and α-tubulin antibodies and 4,6-diamidino-2-phenylindole (DAPI) for the analysis by immunofluorescence microscopy. Representative examples of siRNA MM- and siRNA Plk1-transfected keratinocytes are depicted. The mitotic index and the percentage of cells with aberrant mitotic spindles were determined by counting 250–300 cells (means±s.d.,n=5, for each sample of cells). Scale bar, 5 μm. (e) Plk1-depleted keratinocytes were labelled using BubR1 and α-tubulin antibodies and DAPI for the analysis by immunofluorescence microscopy. Representative examples of Plk1-transfected keratinocytes in different mitotic stages are depicted. Scale bar, 5 μm. Figure 4: Effect of Plk1 silencing on the cell-cycle distribution of primary mammalian cells. Primary cells ( a ) HUVEC and ( b ) fibroblasts and ( c ) keratinocytes were transfected with siRNA MM or siRNA Plk1 at different concentrations (50–100 nM) and analysed by FACS at 24 and 48 h. Representative histograms and the quantification of the cell-cycle analysis are shown. ( d ) Keratinocytes were labelled using Plk1, pericentrin and α-tubulin antibodies and 4,6-diamidino-2-phenylindole (DAPI) for the analysis by immunofluorescence microscopy. Representative examples of siRNA MM- and siRNA Plk1-transfected keratinocytes are depicted. The mitotic index and the percentage of cells with aberrant mitotic spindles were determined by counting 250–300 cells (means±s.d., n =5, for each sample of cells). Scale bar, 5 μm. ( e ) Plk1-depleted keratinocytes were labelled using BubR1 and α-tubulin antibodies and DAPI for the analysis by immunofluorescence microscopy. Representative examples of Plk1-transfected keratinocytes in different mitotic stages are depicted. Scale bar, 5 μm. Full size image Considering the critical roles of polo and its homologues for the formation of an intact spindle apparatus in Drosophila and human cells [35] , [36] , we analysed the spindle structures of Plk1-depleted cells using anti-α-tubulin and -pericentrin mAbs for immunofluorescence staining. In a Plk1-depleted HeLa cell population, 31% of the cells displayed bipolar and 69% aberrant mitotic spindles (mostly monopolar spindles) associated with diffuse spindle pole morphology in the majority of cells ( Supplementary Fig. S4c ). In contrast, an equal level of Plk1 depletion in keratinocytes induced aberrant mitotic spindles in only 14.2% of the cells associated with a mitotic index of 7.5% compared with 0.47% in the siRNA MM-treated cells ( Fig. 4d ). Taken together, Plk1 silencing induced mitotic arrest accompanied by spindle defects in primary cells at a much lower frequency than those of different types of cancer cells. Assessment of apoptosis following Plk1 silencing To determine whether the mitotic delay is caused by chronic activation of the SAC resulting in cell death [37] , [38] , [39] , we analysed whether BubR1 was localized to kinetochores, because unattached kinetochores are associated with several checkpoint proteins, including BubR1. In a high percentage of kinetochores in mitotic Plk1-depleted HeLa cells, BubR1 was enriched at the kinetochores (94.8%: 74/78), even in cells with a metaphase-like phenotype ( Supplementary Fig. S4d ). In contrast, in Plk1-depleted keratinocytes, BubR1 was frequently found on kinetochores in prometaphase, but not in metaphase ( Fig. 4e ). The ability of Plk1 RNAi keratinocytes to enter anaphase may therefore correlate with the lack of SAC activation. Next, we evaluated the correlation between Plk1 silencing and death initiation. In a small collection of cancer cells, the death sensitivity following Plk1 depletion varied considerably ( Supplementary Fig. S5a–e ). The RNAi-mediated iKD50 Plk1− -induced apoptosis in siRNA Plk1-treated cancer cells was between 1.1- and 7.6-fold higher compared with the apoptosis of the siRNA MM-treated cells (iKD50 Plk1− HeLa: 2.0× relative (rel.) apoptosis; MDA-MB-231: 1.5×; SW480: 7.6×; and SK-OV-3: 1.1×; 293T: 2–3×; Supplementary Fig. S5a–e , Table 1 ). Remarkably, the viability of the primary cells was robust on Plk1 depletion; in ES cells, a crucial reservoir for hematopoietic differentiation, the indications of apoptosis induction were weak ( Fig. 5a ). Despite a half-maximal depletion of the Plk1 protein, only relatively low levels of apoptosis were induced in the primary cells (iKD50 Plk1− HUVEC: 1.3× rel. apoptosis; fibroblasts: 1.2×; and keratinocytes: 1.3×; Figs 5b–d , 3a , Table 1 ). 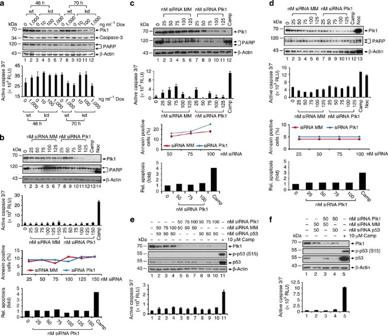Figure 5: Assessment of apoptosis in Plk1-depleted primary mammalian cells. (a) (Upper) Correlation of the Dox (0–1,000 ng ml−1)-induced knockdown of the Plk1 protein and the induction of apoptosis in lysates of wt and transgenic ES cells treated with Dox for 46 or 70 h are shown. The immunoblot for Plk1, caspase-3, PARP and β-actin is also presented. (Lower) Caspase-3 activity was determined in the cell lysates using the Caspase-Glo 3/7 Assay (means±s.d.,n=3, for each concentration). (Upper) Lysates of Plk1 siRNA-transfected (b) HUVEC, (c) fibroblasts and (d) keratinocytes were immunoblotted for Plk1, PARP and β-actin. Camptothecin (Camp) and/or nocodazole (Noc) controls are included. (Middle) Caspase-3 activity was determined in the cell lysates using the Caspase-Glo 3/7 Assay (means±s.d.,n=3, for each concentration). (Lower) Annexin V-based measurements of cells treated with siRNA Plk1 or a siRNA control (siRNA MM) were correlated with levels of apoptosis. (Upper) Lysates of siRNA (Plk1 and/or p53)-transfected (e) keratinocytes and (f) HUVEC cells were immunoblotted for Plk1, p53, p-p53(S15) and β-actin. Camptothecin (Camp) controls are included. (Lower) Caspase-3 activity was determined in the cell lysates using the Caspase-Glo 3/7 Assay (means±s.d.,n=3, for each concentration). Figure 5: Assessment of apoptosis in Plk1-depleted primary mammalian cells. ( a ) (Upper) Correlation of the Dox (0–1,000 ng ml −1 )-induced knockdown of the Plk1 protein and the induction of apoptosis in lysates of wt and transgenic ES cells treated with Dox for 46 or 70 h are shown. The immunoblot for Plk1, caspase-3, PARP and β-actin is also presented. (Lower) Caspase-3 activity was determined in the cell lysates using the Caspase-Glo 3/7 Assay (means±s.d., n =3, for each concentration). (Upper) Lysates of Plk1 siRNA-transfected ( b ) HUVEC, ( c ) fibroblasts and ( d ) keratinocytes were immunoblotted for Plk1, PARP and β-actin. Camptothecin (Camp) and/or nocodazole (Noc) controls are included. (Middle) Caspase-3 activity was determined in the cell lysates using the Caspase-Glo 3/7 Assay (means±s.d., n =3, for each concentration). (Lower) Annexin V-based measurements of cells treated with siRNA Plk1 or a siRNA control (siRNA MM) were correlated with levels of apoptosis. (Upper) Lysates of siRNA (Plk1 and/or p53)-transfected ( e ) keratinocytes and ( f ) HUVEC cells were immunoblotted for Plk1, p53, p-p53(S15) and β-actin. Camptothecin (Camp) controls are included. (Lower) Caspase-3 activity was determined in the cell lysates using the Caspase-Glo 3/7 Assay (means±s.d., n =3, for each concentration). Full size image As p53-deficient cancer cells were more sensitive to Plk1 inhibition than cells with functional p53 (refs 40 , 41 ), we evaluated the involvement of p53 status in apoptosis induced by Plk1 silencing in primary cells. Although the levels of Plk1 and p53 were efficiently depleted in keratinocytes and HUVEC, apoptosis was not apparent, suggesting a different role of the p53 for the sensitivity of certain primary cells towards Plk1 inhibitors ( Fig. 5e,f ). Assessing the effects of the Plk1 inhibitor BI 2536 in MEFs Remarkably, the treatment of MEFs with the small molecule inhibitor BI 2536 (25–250 nM) revealed a pronounced growth inhibition at elevated concentrations ( Fig. 6a ), which was also reflected by the cell-cycle profile ( Fig. 6b ) at decreasing Plk1-specific kinase activities ( Fig. 6c ). The incubation with 50 nM BI 2536 induced aberrant mitotic spindles in 78% of MEFs associated with a mitotic index of >7.0% compared with control cells ( Fig. 6d ). As the EC 50 values for BI 2536 in primary cells were reported to be 12–31 nM (ref. 42 ), we evaluated the induction of apoptosis in an extended range of concentrations (10 nM–2 μM; Fig. 6e,f ). In contrast to the small extent of siRNA-induced apoptosis, BI 2536 treatment increased the level of apoptosis considerably in MEFs up to 20–30% annexin-positive cells at concentration ≥100 nM ( Fig. 6e,f ). 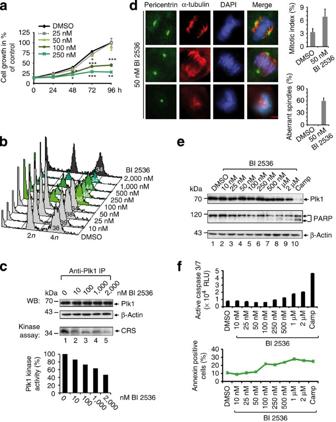Figure 6: Assessment of cell-cycle properties and apoptosis in BI 2536-treated MEFs. (a) Proliferative activity of MEFs at different BI 2536 concentrations (25–250 nM; means±s.d.,n=3, for each concentration). *P<0.05, **P<0.01, ***P<0.001, Student'st-test, unpaired and two-tailed. (b) FACS profile of exponentially growing MEFs treated for 24 h with BI 2536 (10 nM–2 μM). Percentage of cells in G2/M are given at each concentration. (c) Kinase activity of immunoprecipitated Plk1 protein from MEFs treated for 24 h with BI 2536 (10 nM–2 μM) using the cytoplasmic retention signal (CRS) of cyclin B1 as substrate. (d) MEFs were labelled using Plk1, pericentrin and α-tubulin antibodies and 4,6-diamidino-2-phenylindole for the analysis by immunofluorescence microscopy. Representative examples of BI 2536-treated and control MEFs are depicted. Scale bar, 5 μm. The mitotic index and the percentage of cells with aberrant mitotic spindles were determined by counting 250–300 cells (means±s.d.,n=5, for each sample of cells). (e) The correlation of BI 2536-mediated inhibition of the Plk1 and the induction of apoptosis in MEFs was analysed. The immunoblot for Plk1, β-actin and PARP is presented. (f) Annexin V-based measurements and caspase activity were determined in cell lysates of BI 2536-treated MEFs (24 h) using the Caspase-Glo 3/7 Assay (means±s.d.,n=3, for each concentration). Figure 6: Assessment of cell-cycle properties and apoptosis in BI 2536-treated MEFs. ( a ) Proliferative activity of MEFs at different BI 2536 concentrations (25–250 nM; means±s.d., n =3, for each concentration). * P <0.05, ** P <0.01, *** P <0.001, Student's t -test, unpaired and two-tailed. ( b ) FACS profile of exponentially growing MEFs treated for 24 h with BI 2536 (10 nM–2 μM). Percentage of cells in G 2 /M are given at each concentration. ( c ) Kinase activity of immunoprecipitated Plk1 protein from MEFs treated for 24 h with BI 2536 (10 nM–2 μM) using the cytoplasmic retention signal (CRS) of cyclin B1 as substrate. ( d ) MEFs were labelled using Plk1, pericentrin and α-tubulin antibodies and 4,6-diamidino-2-phenylindole for the analysis by immunofluorescence microscopy. Representative examples of BI 2536-treated and control MEFs are depicted. Scale bar, 5 μm. The mitotic index and the percentage of cells with aberrant mitotic spindles were determined by counting 250–300 cells (means±s.d., n =5, for each sample of cells). ( e ) The correlation of BI 2536-mediated inhibition of the Plk1 and the induction of apoptosis in MEFs was analysed. The immunoblot for Plk1, β-actin and PARP is presented. ( f ) Annexin V-based measurements and caspase activity were determined in cell lysates of BI 2536-treated MEFs (24 h) using the Caspase-Glo 3/7 Assay (means±s.d., n =3, for each concentration). Full size image Evaluation of the tumour regression activity of Plk1-iKD When transplanted into an ectopic location in athymic animals, ES cells can develop into tumours that are called teratocarcinomas [43] . Here, we compared Plk1- and Luc-iKD ES cells in vivo to determine the role of Plk1 during tumour development of primary cells. The Dox-induced reduction of Plk1 mRNA and protein in Plk1- and Luc-iKD ES cells was investigated ( Fig. 7a ). The injection of Plk1-iKD ES cells into the right flank and the Luc-iKD ES cells into the left flank of the same athymic mouse provided a side-by-side comparison in the presence or absence of Dox. Although the growth behaviour of the non-induced Plk1-, Luc-iKD ES cells and the Dox-induced Luc-iKD ES cells did not differ significantly, 38 days after inoculation Dox-treated animals carrying Plk1-iKD ES cell-derived teratocarcinomas exhibited a significant growth reduction of more than 82% ( P <0.05, Student's t -test) compared with the control ( Fig. 7b,c ). The subsequent protein analysis of tumour tissues (±Dox) confirmed the prominent depletion of Plk1 in Dox-induced Plk1-iKD ES cell-derived tumours ( Fig. 7d ). Our data strongly suggest that the inhibition of tumour growth derived from primary cells correlates to Plk1 depletion. 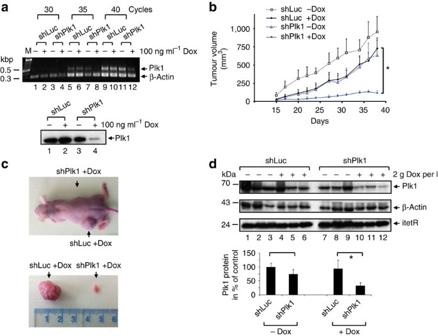Figure 7: Assessment of growth properties of ES cell-derived teratocarcinomas. (a) Plk1 mRNA and protein levels in Plk1-iKD- and Luc-iKD-ES cells (±Dox) determined by semi-quantitative RT-PCR analysis and western blot. (b) Volumes of teratocarcinomas derived from Plk1-iKD- and Luc-iKD-ES cells (inoculated on opposite flanks of the same animal) either after induction with Dox or in the absence of Dox starting with 3 days before inoculation. Significant inhibition of tumour growth (P<0.05) is indicated with an asterisk (means±s.d.,n=12, for each time point). (c) Representative image of a mouse exhibiting Plk1-iKD- and Luc-iKD-ES cell-derived tumour growth on opposite flanks. (d) Total cellular protein was prepared from Plk1-iKD- and Luc-iKD-ES cell tumours and separated by SDS–PAGE for anti-Plk1, -itetR and -β-actin immunoblotting analyses (means±s.d.,n=3, for each treatment). *P<0.05, Student'st-test, unpaired and two-tailed. Figure 7: Assessment of growth properties of ES cell-derived teratocarcinomas. ( a ) Plk1 mRNA and protein levels in Plk1-iKD- and Luc-iKD-ES cells (±Dox) determined by semi-quantitative RT-PCR analysis and western blot. ( b ) Volumes of teratocarcinomas derived from Plk1-iKD- and Luc-iKD-ES cells (inoculated on opposite flanks of the same animal) either after induction with Dox or in the absence of Dox starting with 3 days before inoculation. Significant inhibition of tumour growth ( P <0.05) is indicated with an asterisk (means±s.d., n =12, for each time point). ( c ) Representative image of a mouse exhibiting Plk1-iKD- and Luc-iKD-ES cell-derived tumour growth on opposite flanks. ( d ) Total cellular protein was prepared from Plk1-iKD- and Luc-iKD-ES cell tumours and separated by SDS–PAGE for anti-Plk1, -itetR and -β-actin immunoblotting analyses (means±s.d., n =3, for each treatment). * P <0.05, Student's t -test, unpaired and two-tailed. Full size image Despite their proven clinical success in the treatment of cancer patients, tubulin agents, such as taxanes or vinca alkaloids, affect normal cells and cause clinical symptoms including myelosuppression and neuropathies [5] . Thus, to minimize these side effects, non-structural components of mitosis have become the focus of potential drugs. Recent exploration of mitotic progression has identified critical effectors (kinesins, Aurora kinase, Plk1), all of which are drug-target classes [5] . The successful validation of Plk1 as a drug target based on its analysis in cancer cell lines in vitro and in vivo led to the rapid pharmaceutical development and clinical evaluation of a growing number of Plk inhibitors. Still, a major concern in targeting Plk1 for cancer therapy is the potential toxicity in normal tissues due to the pleiotropic functions of Plk1 in mitosis [44] . However, data on the role of Plk1 in primary and primary-like cells are rare and controversial: although the inhibition of Plk1 by antibody microinjection or with the small molecule inhibitor BI 2536 induced G 2 or mitotic arrest, respectively, in both of these studies, the apoptotic response was not determined [36] , [42] . A recent analysis describes a differential effect of BI 2536 on the proliferative activity of primary cardiomyocytes and cardiac fibroblasts [45] . In contrast, Plk1 depletion in a nontransformed retinal epithelial cell line that stably expresses human telomerase reverse transcriptase (hTERT-RPE1) only had a minor effect on the kinetics and percentage of cells that enter and exit from mitosis [41] . Given that the immortalization of epithelial cells due to the expression of hTERT is accompanied by genetic and/or epigenetic alterations, the extent to which these cells reflect primary cells is unknown [46] . Thus, because the Plk1-knockout mice were not viable [17] , we decided to investigate the putative toxicities of Plk1 silencing in a GEMM. Although anti-mitotics such as Taxol or hypomorphic alleles of the Drosophila polo gene lead to disorders of spermatogenesis [47] , [48] , the testes, which exhibited the most pronounced iKD, lacked histological and functional abnormalities. In summary, our data suggest that an efficient, but not complete, knockdown of Plk1 in primary murine cells embedded in the microenvironment of their corresponding organs has only a minor physiological impact on the functions analysed like the proliferative activity. In our study, we extended our examination to primary cells in cell culture to determine whether the tissue context is critical for the dependence on Plk1 and whether the responses of primary cells to Plk1-depletion under controlled cell culture conditions are reflected in the Plk1-iKD mice. The toxicity of Plk1 depletion suggested a model in which cancer cells of different origin, regardless of the transforming oncogenic mechanism, are often addicted to Plk1. Notably, primary cells (even those removed from their normal microenvironment) are largely resistant to apoptosis by low levels of Plk1, suggesting their weak dependence on Plk1 (non-addiction), which correlates with normal spindle dynamics and low SAC activities. Hence, our study suggests the existence of a therapeutic window for monospecific Plk1 inhibitors to kill tumour cells while sparing normal cells. This differential addiction of normal and cancer cells to Plk1 may also provide the rationale for using Plk1-monospecific drugs for chemoprevention in individuals with a hereditary cancer background (for example, breast, colon and prostate) or in other patients with premalignant lesions such as ductal carcinoma in situ DCIS. Clinical trials have revealed that the Plk1 inhibitor BI 2536 exhibits anti-tumour activity in patients, and reversible neutropenia was the main dose-limiting toxicity [49] , [50] . Plk1-iKD mice did not provide evidence for significant haematological alterations, although reduced ferritin levels indicate a depletion of iron stores that could induce hematopoietic abnormalities [29] . Obvious differential effects between the clinical trials and our iKD model could be due to mechanistic differences of the siRNA and small molecule inhibitors. Whether the gradual depletion of Plk1 by RNAi allows primary cells with intact checkpoints to activate compensatory pathways involving related kinases remains to be explored. The expression of other representatives of the Plk family in Plk1-depleted cells and tissues opens the possibility of a substitutable role by other family members. Notably, ATP-competitive inhibitors of Plk1, such as PHA-680626 and BI 2536, scarcely discriminate between Plk1 and Plk3, because the residues that line the ATP-binding pocket are highly conserved within the Plk family except Plk4 (ref. 16 ). This simultaneous inhibition of different Plks including Plk1 might intensify the apoptotic response of primary cells as observed here in BI 2536-treated MEFs. Although more predictive models are urgently required in cancer drug development, GEMMs are not yet an integral part of pharmacological research. Inducible RNAi-based GEMMs provide a unique opportunity to reversibly control gene expression in different tissues of adult mice and to study responses to a target-specific KD. Our study represents an attempt to assess the feasibility of using inducible RNAi-based GEMMs to predict the toxicities of targeted cancer drugs in mice. The similarities in KD responses observed in our Plk1-iKD mice and in our siRNA-treated primary cells validated the preclinical and predictive utility of iKD GEMMs in providing information on potential mechanism-based toxicities that might arise as a result of the pharmacological inactivation of Plk1. Isolation of total RNA from murine tissues After Dox-treatment wt and Plk1-iKD mice were rapidly killed. Organs were prepared and stored in RNAlater Stabilization Reagent (Qiagen). For the RNA preparation, tissue pieces of 20 mg were dispersed with a PCR Tissue Homogenizing Kit (Omni International). Then total RNA was isolated using an RNeasy Mini Kit (Qiagen). The RNA was stored at concentrations of 50 ng μl −1 to 1 μg μl −1 at −20 °C. Plk1 expression analysis For northern blot experiments, 2 μg poly(A) + RNA was subjected to 1.5% denaturating agarose gel-electrophoresis. The RNA was blotted to a Hybond-N+ nitrocellulose membrane (Amersham Biosciences) overnight by capillary forces. Subsequently, the membranes were heated at 80 °C (2 h) to fix the RNA. The mRNA (Plk1, β-actin) was hybridized using a radioactive probe-containing α-[P 32 ]-dCTP (1×10 6 c.p.m. ml −1 ). Probes for detecting the Plk1 mRNA were generated by standard PCR protocols using the sense primer 5′-TAATGACTCAACACGCCTGATT-3′ and the antisense primer 5′-AGCTCAGCAGCTTGTCTACCAT-3′. The β-actin-specific probe was generated using the sense primer 5′-GAGGAGCACCCCGTGCTGCTGACCGAGGCC-3′ and the antisense primer 5′-CCTGCTTGCTGATCCACATCTGCTGGAAGGTG-3′. To quantify Plk1 transcripts, 1 μg of RNA was subjected to qRT-PCR (High Capacity cDNA Reverse Transcription Kit, Applied Biosystems). The qRT-PCR was conducted using a TaqMan Gene Expression Assay for murine Plk1 (Applied Biosystems). As an internal control in the TaqMan Assay, murine β-actin was used (Applied Biosystems). Real-time PCR This assay was performed using a standard TaqMan PCR Kit protocol in Applied Biosystems Step One. The 10 μl PCR reaction included 0.67 μl RT product, 1× TaqMan Universal PCR Master Mix, 0.2 μM TaqMan probe, 1.5 μM forward primer and 0.7 μM reverse primer. The reactions were incubated in a 384-well plate at 95 °C (10 min), followed by 40 cycles of 95 °C (15 s) and 60 °C (1 min). All reactions were run in triplicate. Preparation of primary cells and cell culture MEFs were prepared from 15-day-old embryos by a standard procedure [51] . Splenocytes and bone marrow cells were isolated by standard protocols [51] , [52] . For Dox-treatment ES cells were cultured in DMEM (Invitrogen) containing 10% FCS from PAA, 4,500 mg l −1 glucose, 1× non-essential amino acids and various concentrations of Dox (Sigma). The Dox-medium was prepared and changed each day. For the isolation of HUVEC, an umbilical vein was cannulated with a sterile needle and perfused by PBS to remove remaining blood for subsequent incubation with α-chymotrypsin (Sigma). The umbilical cord was then flushed with RPMI 1640 medium (Invitrogen). After centrifugation, cells were resuspended and cultured in RPMI 1640 medium with 75 μg ml −1 endothelial cell growth supplement (Sigma). Fibroblasts were cultured in DMEM with 10% FCS and keratinocytes in Dermalife K Medium Complete Kit (Cell Systems) at 37 °C and 5% CO 2 in a humidified environment. Research studies involving the use of human specimens were reviewed and approved by the Institutional Review Board of the Goethe-University School of Medicine. Cancer cell lines were purchased from the American Type Culture Collection and grown in the recommended medium supplemented with 10% FCS at 37 °C and 5% CO 2 in a humidified environment. SW480 (colon), MDA-MB-231 (breast) and 293T (kidney/embryonic +T) cells were grown in DMEM, HeLa (cervix) cells in MEM and SK-OV-3 (ovarian) cells in McCoy's 5a. Media were obtained from Invitrogen and McCoy's was from Biochrom. Transfections One day before transfection, 2×10 5 Art4.12 ES cells carrying the FRT/F3 configuration at rosa26 were plated on a 3-cm dish in 2 ml medium [20] . Before transfection 2 ml fresh medium was added. A volume of 3 μl FuGENE 6 Reagent (Roche) were mixed with 100 μl serum-free medium (OptiMEM 1 with Glutamax-I, Invitrogen) and incubated (5 min). A volume of 100 μl of the FuGENE 6/OptiMEM solution was added to 2-μg circular DNA ( c =0.33 μg μl −1 ) and incubated (15 min). Fresh medium was added to the transfected cells the following day. From day 2 on, the medium was changed daily, replaced by medium containing 250 μg ml −1 G418 (Geneticin, Invitrogen). The siRNA against Plk1 and the control siRNA MM [31] were purchased from Sigma. Normal cells were transfected with siRNA (10–150 nM) using Gene Silencer (BioCat). Cells were collected after 24 or 48 h. The transfection efficiency was ascertained by transfecting FITC-labelled siRNA (6 h) followed by FACS analysis (FACScan, BD Biosciences). Cancer cells were transfected with siRNAs (0.5–10 nM) using the Oligofectamine protocol (Invitrogen). Control cells were treated as indicated for each experiment. Cells were collected 24 h after transfection for western blot, cell-cycle analysis and the apoptosis assay. For cell-cycle kinetics, the HeLa and SW480 cells were collected 0, 3, 6, 9, 12, 15 and 18 h after the addition of siRNAs. Proliferation was measured 0, 24, 48, 72 and 96 h after siRNA transfection. Synchronization Cells were incubated with 2 mM thymidine (Sigma; 16 h), washed extensively with PBS and released in fresh medium (8 h), followed by a second thymidine block (16 h) [12] . Investigating the cell-cycle distribution by FACS analysis Cells were seeded, transfected and collected after 24 and 48 h or every 3 h for the cell-cycle kinetics. Cells were trypsinized, washed with PBS and fixed in 70% ice-cold ethanol (30 min). After centrifugation, the cells were resuspended in PBS and incubated with 300 μg ml −1 RNAse A and 30 μg ml −1 propidium iodide (30 min) at 37 °C. Finally, the cell-cycle quantification was performed by flow cytometry (FACScan, BD Biosciences) using ModFit (Verity Software House). Immunofluorescence assays Cells were grown on a glass coverslip, fixed and permeabilized with methanol (−20 °C), and washed with PBS before the addition of appropriate primary and secondary antibodies. Microscopy was performed using a Zeiss Axio Imager.Z1 microscope (Zeiss) equipped with a ×40 objective, and the images were captured and processed using AxioVision Software (Zeiss). Analysis of apoptosis The Vybrant Apoptosis Assay Kit no. 2 (Alexa Fluor 488 annexin V/propidium iodide staining, Invitrogen) was used, and the cells were analysed by flow cytometry using a FACScan (BD Biosciences) [53] . The activity of caspase-3/7 was determined using the Caspase-Glo 3/7 Assay according to the manufacturer's instructions (Promega). Antibodies The following antibodies were used: mouse monoclonal antibodies against Plk1 (1:1,000), Cdk1 (1:1,000), cyclin B1 (1:5,000), p53 (1:2,000; Santa Cruz), Plk2 (1:500), β-actin (1:200,000; Sigma), Plk3 (1:1,000; BD Pharmingen), α-tubulin (1:500,000; Cedarlane/Biozol), Emi1 (1:500; Invitrogen, Karlsruhe), Securin (1:1,000; Abcam) and Ki-67 (1:100; DAKO), and rabbit polyclonal antibodies against PARP (1:1,000), Plk4 (1:1,000; Cell Signaling Technology/New England Biolabs), GAPDH (1:1,000; Abcam), Plk1 (1:1,000), pericentrin (1:500), caspase-3 (1:1,000), phospho-p53(Ser15) (1:500; Cell Signaling Technology/New England Biolabs), tet-Repressor (1:5,000; MoBiTec/Invitrogen), phospho-Histone H3(S10) (1:1,000; Millipore), and phospho-Cdk1 (T14/Y15) (1:1,000; Santa Cruz), which were obtained from commercial sources. HRP-conjugated secondary antibodies (1:5,000) were from Santa Cruz; conjugated antibodies to FITC, CY3 and CY5 (1:1,000) were obtained from Jackson Immuno Research Labs; and biotinylated secondary antibodies were from DAKO. Cell proliferation assay Cell viability and proliferation assays were conducted using the CellTiter-Blue Cell Viability Assay (Promega). Cells were seeded in 96-well plates and siRNA transfected or BI 2536 treated, and after 0, 24, 48, 72 or 96 h, the fluorescence was measured using a Victor 1420 Multilabel Counter (Wallac/PerkinElmer). Statistical methods The mean mRNA levels measured by qRT-PCR were calculated using the averages of at least five independent samples. All other experiments were performed at least in triplicate. Mouse data depicted in Supplementary Table S2 and S5 were determined by two-way ANOVA, all other assays were analysed by Student's t -test, unpaired and two-tailed. Significant differences are indicated with stars (* P <0.05, ** P <0.01, *** P <0.001). Tumour mouse model Each flank of 8-week-old female athymic mice (Harlan-Winkelmann) was inoculated subcutaneously with 2×10 6 ES cells resuspended in 0.25 ml sterile saline solution. Luc-iKD ES cells were inoculated on the left flank, whereas Plk1-iKD ES cells were inoculated on the right flank. Mice were distributed randomly into two groups (12 animals each) for the subsequent analysis of tumour development with and without Dox-treatment. Dox (Sigma) was applied as 0.2% solution in the drinking water with additional 3% sucrose dissolved in natural mineral water starting 2 days after inoculation. Drinking water for control mice contained 3% sucrose without Dox. Tumours (teratocarcinomas) were measured in two right-angled dimensions by a sliding caliper three times a week. Absolute tumour volumes were evaluated according to V (mm 3 )=π/6 ab 2 with a > b . After inoculation measurements started at day 7 and finished at day 38 followed immediately by killing the animals. Three individual tumours from all four groups (Luc-iKD- and Plk1-iKD-ES cells, ±Dox) were analysed. The use of animals complied with the regulations of the Goethe-University. Additional methods Specific reagents and methodology for the inducible shRNA expression vector (exchange vector), generation of ES cells, mice, analysis of mouse genotypes, stem–loop RT-PCR, western blot, pathology screen, immunohistochemistry, collection and analysis of blood samples are all described in the Supplementary Methods . How to cite this article: Raab, M et al . Toxicity modelling of Plk1-targeted therapies in genetically engineered mice and cultured primary mammalian cells. Nat. Commun. 2:395 doi: 10.1038/ncomms1395 (2011).